LRRC19 expressed in the kidney induces TRAF2/6-mediated signals to prevent infection by uropathogenic bacteria The innate immune-dependent bactericidal effects are critical for preventing microbial colonization in the urinary system. However, the mechanisms involved in establishing innate immune responses in kidney are not completely understood. Here we describe the role of a novel member of the LRR (leucine-rich repeat) class of transmembrane proteins, LRRC19 (LRR-containing 19) in eliminating uropathogenic bacteria. LRRC19 is predominantly expressed in human and mouse kidney tubular epithelial cells and LRRC19-deficient mice are more susceptible to uropathogenic Escherichia coli (UPEC) infection than wild-type or TLR4 knockout mice. Recognition of UPEC by LRRC19 induces the production of cytokines, chemokines and antimicrobial substances through TRAF2- and TRAF6-mediated NF-κB and MAPK signalling pathways. Thus, LRRC19 may be a critical pathogen-recognition receptor in kidney mediating the elimination of UPEC infection. Renal bacterial infections are common infectious diseases that can impair renal function and/or lead to renal tubulointerstitial nephritis. These urinary tract infections (UTIs) are most commonly caused by uropathogenic Escherichia coli (UPEC) [1] , [2] . UPEC can invade kidney tissue and specifically bind to the apical surface of collecting duct cells [3] . However, in healthy individuals, kidneys remain free from microbial colonization. Innate immune-dependent bactericidal effects in the kidney are a critical mechanism for preventing bacterial infection. Renal epithelial cells are the first to encounter ascending pathogens and respond to microbial challenge by initiating inflammatory responses. The generated proinflammatory mediators such as TNF-α (tumour necrosis factor-alpha), IL-6 (interleukin-6), MCP-1 (monocyte chemotactic protein-1) and MIP-2 (macrophage inflammatory protein 2), can recruit inflammatory cells including monocytes and neutrophils to kidney tissue to kill the bacterial cells [4] , [5] . Kidney epithelial cells also produce antimicrobial peptides and proteins, including defensins such as β-defensin-1 (ref. 6 ), β-defensin-3 (ref. 7 ), α-defensin-5 (ref. 8 ) and cathelicidins [9] . In addition, C-type lectins such as Reg3 are also found in the epithelial cells [10] . All of these are important in eliminating UPEC from the kidney. However, the mechanisms involved in orchestrating the expression of these inflammatory factors are not completely understood. Inflammatory mediators are largely modulated by pathogen-recognition receptors (PRRs). Most of these PRRs are LRR proteins, which constitute a prominent extracellular family [11] . Multiple classes of PRRs such as Toll-like receptors (TLRs) have been identified as important components of innate immunity, participating in the sensory system for host defense against the invasion of infectious agents. Murine renal tubular epithelial cells express multiple TLRs, including TLR1, 2, 3, 4, 6 and 11 (ref. 12 ). These TLRs are involved in preventing infection by both Gram-negative and Gram-positive pathogenic bacteria by modulating the expression of inflammatory cytokines, chemokines and antimicrobial peptides and proteins [13] . For example, TLR4, which recognizes lipopolysaccharide (LPS), the main component of Gram-negative bacterial cell wall, induces the inflammatory responses to UPEC [14] . In animal models, TLR2 (ref. 15 ), TLR4 (ref. 14 ), TLR5 (ref. 5 ) and TLR11 (ref. 16 ) also regulate susceptibility to UTIs. In addition, several studies in humans also indicate the association of TLR2 and TLR4 polymorphisms with UTI [17] . Similar to the immune cells such as dendritic cells [18] , [19] , medullary collecting duct cells produce inflammatory responses to UPEC via TLR4-mediated MyD88 (myeloid differentiation factor 88)-dependent NF-κB and MAPK (mitogen-activated protein kinases) pathways [12] . However, UPEC also induce inflammatory responses via a TLR4 -independent and MyD88-independent pathways [12] . Typically, renal collecting duct epithelial cells may be activated through TNF receptor-associated factor 2 (TRAF2)—and TNF receptor-associated factor 6 (TRAF6)-dependent, but not MyD88-dependent signalling pathways [3] . Thus, different kinds of pathogen-recognition receptors and signalling pathways may be involved in inflammatory responses against UPEC. Here, we identified a novel class of pathogen-recognition receptor, LRR-containing 19 (LRRC19), which is predominantly expressed in human and mouse kidney tissues and involved in the clearance of UPEC. We offer evidence that LRRC19 can recognize UPEC and activate NF-κB and MAPK to induce production of proinflammatory cytokines, chemokines and antimicrobial substances in kidney tubular epithelial cells. Data also indicate that LRRC19-induced inflammatory responses occur through TRAF2 and TRAF6-mediated signalling pathways. LRRC19 promotes UPEC elimination by kidneys Our previous data indicate that LRRC19-transfected human embryonic kidney (HEK) 293T cells can produce an inflammatory response to multiple TLR ligands such as LPS [20] , suggesting that LRRC19 may act as a pathogen-recognition receptor. To further investigate the roles of LRRC19 in defending against infection, we generated LRRC19-deficient ( Lrrc19 KO ) mice by homologous recombination technique ( Supplementary Fig. 1 ). Phenotype analysis showed that the Lrrc19 KO mice did not show abnormalities in the populations and surface molecules of immune cells as compared with their wild-type (WT) littermates. As LRRC19 was strongly expressed in mouse and human kidney tissue, especially renal collecting duct epithelial cells [20] ( Fig. 1a,b and Supplementary Fig. 2 ), LRRC19 might have a specific role in inducing innate immune responses against UPEC infection. Thus, we first examined the susceptibility of Lrrc19 KO mice to infection by UPEC. WT and Lrrc19 KO mice were transurethrally inoculated with 5.0 × 10 7 clone-forming units (CFU) of UPEC CFT073. No significant differences in bacterial counts were observed between WT and Lrrc19 KO mice in the kidney at day 1. However, at 3 days post inoculation, more bacteria, with a median of 1.3 × 10 3 CFU per gram tissue, were found in Lrrc19 KO kidney tissue than in WT kidney tissue with a median bacterial load of 7.1 × 10 2 CFU per gram kidney tissue ( P <0.001) ( Fig. 1c ). Until 7 days post infection, Lrrc19 KO mice still had a median of 1.1 × 10 2 CFU per gram kidney tissue; whereas no bacteria were detected in WT kidney tissue ( Fig. 1c ). In addition, bacteria were also often detected in the livers of UPEC-infected Lrrc19 KO mice but not in WT mice. Notably, in each case, the bladder was almost equally infected by UPEC in WT and Lrrc19 KO mice ( Fig. 1c ), indicating a tissue-specific effect of LRRC19 in the kidney. We also assessed the intrinsic function of hematopoietic cells or renal epithelial cells in eliminating UPEC. WT/WT (WT bone marrow (BM) donor cells into lethally irradiated WT recipients) but not KO / KO ( Lrrc19 KO BM donor cells into lethally irradiated Lrrc19 KO recipients) chimeras could effectively eliminate UPEC from kidney tissue ( Fig. 1d ), further confirming the functional potential of LRRC19 in preventing UPEC infection. Notably, more bacteria were found in WT/ Lrrc19 KO (WT BM donor cells into lethally irradiated Lrrc19 KO recipients) kidney tissue and in Lrrc19 KO /WT ( Lrrc19 KO BM donor cells into lethally irradiated WT recipients) kidney tissue than in WT/WT kidney tissues ( P <0.01; Fig. 1d ), suggesting that both kidney cells and hematopoietic cells are important for LRRC19-mediated elimination of UPEC in kidney. Supporting this conclusion, LRRC19 could also be detected in CD11b positive cells (neutrophils) from the spleen, which are important effectors in the defense against UPEC. Taken together, LRRC19 have a role in eliminating uropathogenic bacteria in kidney by both hematopoietic cells and renal epithelial cells. 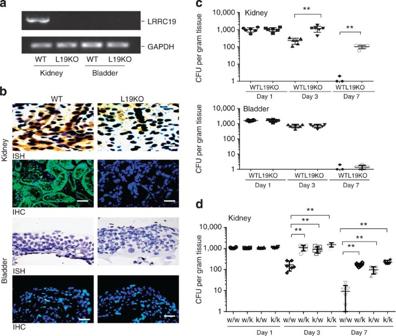Figure 1:Lrrc19 KOmice have reduced ability to eliminate UPEC. (a) RT–PCR analyses of LRRC19 mRNA in the kidney and bladder of WT andLrrc19 KO(L19KO) mice. (b)In situhybridization and immunostaining of LRRC19 in the kidney and bladder of WT andLrrc19 KO(L19KO) mice.In situhybridization (ISH) and immunostaining (IHC) were performed according to the protocol described in the methods. Brown colour and green colour indicated positive staining. Scale bars, 20 μm. (c) Bacterial counts in the kidney and bladder of UPEC-infected WT andLrrc19 KO(L19KO) mice. Kidneys and bladders were removed at day 1, 3 and 7 post infection and homogenates were plated on LB agar to enumerate the CFU per gram of tissue. Colony counts were averaged from three plates per mouse. (d) Bacterial counts in the kidney of chimeric mice at day 1, 3 and 7 post infection. Chimeric mice ofLrrc19 KOand WT C57BL/6 mice were generated by irradiatingLrrc19 KOor WT GFP transgenic C57BL/6 mice and then injecting bone marrow cells obtained from the femurs of donor mice. W/W indicates that bone marrow (BM) cells of WT mice were transplanted into lethally irradiated WT mice; W/K indicates BM cells of WT mice into lethally irradiatedLrrc19 KOmice; K/W indicates BM cells ofLrrc19 KOmice into lethally irradiated WT mice; K/K indicates BM cells ofLrrc19 KOmice into lethally irradiatedLrrc19 KOmice. *P<0.05 and **P<0.01 (Mann–WhitneyUtest incandd). The data are representative of at least three independent experiments. Figure 1: Lrrc19 KO mice have reduced ability to eliminate UPEC. ( a ) RT–PCR analyses of LRRC19 mRNA in the kidney and bladder of WT and Lrrc19 KO (L19KO) mice. ( b ) In situ hybridization and immunostaining of LRRC19 in the kidney and bladder of WT and Lrrc19 KO (L19KO) mice. In situ hybridization (ISH) and immunostaining (IHC) were performed according to the protocol described in the methods. Brown colour and green colour indicated positive staining. Scale bars, 20 μm. ( c ) Bacterial counts in the kidney and bladder of UPEC-infected WT and Lrrc19 KO (L19KO) mice. Kidneys and bladders were removed at day 1, 3 and 7 post infection and homogenates were plated on LB agar to enumerate the CFU per gram of tissue. Colony counts were averaged from three plates per mouse. ( d ) Bacterial counts in the kidney of chimeric mice at day 1, 3 and 7 post infection. Chimeric mice of Lrrc19 KO and WT C57BL/6 mice were generated by irradiating Lrrc19 KO or WT GFP transgenic C57BL/6 mice and then injecting bone marrow cells obtained from the femurs of donor mice. W/W indicates that bone marrow (BM) cells of WT mice were transplanted into lethally irradiated WT mice; W/K indicates BM cells of WT mice into lethally irradiated Lrrc19 KO mice; K/W indicates BM cells of Lrrc19 KO mice into lethally irradiated WT mice; K/K indicates BM cells of Lrrc19 KO mice into lethally irradiated Lrrc19 KO mice. * P <0.05 and ** P <0.01 (Mann–Whitney U test in c and d ). The data are representative of at least three independent experiments. Full size image LRRC19 promotes inflammatory responses in kidneys We next assessed inflammatory responses in WT and Lrrc19 KO mice infected with UPEC. Bladders and kidneys from WT and Lrrc19 KO mice did not exhibit remarkable inflammation at 1 day post infection ( Supplementary Fig. 3 ). However, at 3 days post infection, histological examination showed a greater inflammatory response only in WT kidneys, as measured by infiltration of leukocytes ( Fig. 2a and Supplementary Fig. 3 ). There also appeared fewer inflammatory cells (Ly6G + Ly6C + neutrophils) in the spleens of infected Lrrc19 KO mice than in those of infected WT mice ( Fig. 2b ). Transurethral inoculation of UPECs also greatly upregulated the expression of TNFα, IL-6, MCP-1 and MIP-2 in the kidney tissues of WT mice but not in those of Lrrc19 KO mice ( Fig. 2c,d ). The higher levels of TNFα, IL-6, MCP-1 and MIP-2 were also detected in sera of infected WT mice as compared with Lrrc19 KO mice ( P <0.05; Fig. 2c ). All of these suggest that LRRC19 is involved in the inflammatory responses of kidney to UPEC. 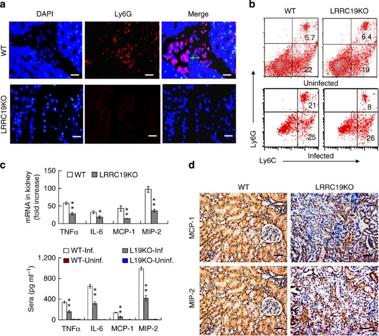Figure 2: LRRC19 deficiency reduces inflammatory responses to UPEC in kidney. (a) Immunostaining observation of the kidney from WT andLrrc19 KOmice at day 3 post infection. 5-μm-thick sections of the infected kidney from WT andLrrc19 KOmice were prepared from frozen tissue. Tissues were stained by PE-labelled anti-Ly6G antibody (Ly6G) and stained by DAPI. Scale bars, 20 μm. (b) Flow cytometry analysis of inflammatory cells. Splenocytes of UPEC-infected WT andLrrc19 KOmice were stained by anti-Ly6G and Ly6C and then analysed by FACScan. Numbers indicate percentage of Ly6G+Ly6C+or Ly6C+cells. (c) qRT–PCR and ELISA of TNFα, IL-6, MCP-1 and MIP-2. TNFα, IL-6, MCP-1 and MIP-2 in the kidney tissues from WT andLrrc19 KOmice 3 days after inoculation with UPEC strain CFT073 were analysed by qRT–PCR (upper). Transcriptional levels of TNFα, IL-6, MCP-1 and MIP-2 were shown as ‘fold increased’ relative to noninfection control. TNFα, IL-6, MCP-1 and MIP-2 in the sera of uninfected (uninf.) and UPEC-infected (Inf.) WT andLrrc19 KO(L19KO) mice were analysed by ELISA (below). (d) Immunostaining analysis of cytokines in the kidney tissues from WT andLrrc19 KOmice 3 days after inoculation with CFT073. Brown colour in immunostaining indicated positive response. Scale bars, 20 μm. *P<0.05 and **P<0.01 (t-test for two groups inc, mean±s.d.; analysis of variance for multiple groups inc, mean±s.e.m.,n=8 mice per group). The data are representative of at least three independent experiments. Figure 2: LRRC19 deficiency reduces inflammatory responses to UPEC in kidney. ( a ) Immunostaining observation of the kidney from WT and Lrrc19 KO mice at day 3 post infection. 5-μm-thick sections of the infected kidney from WT and Lrrc19 KO mice were prepared from frozen tissue. Tissues were stained by PE-labelled anti-Ly6G antibody (Ly6G) and stained by DAPI. Scale bars, 20 μm. ( b ) Flow cytometry analysis of inflammatory cells. Splenocytes of UPEC-infected WT and Lrrc19 KO mice were stained by anti-Ly6G and Ly6C and then analysed by FACScan. Numbers indicate percentage of Ly6G + Ly6C + or Ly6C + cells. ( c ) qRT–PCR and ELISA of TNFα, IL-6, MCP-1 and MIP-2. TNFα, IL-6, MCP-1 and MIP-2 in the kidney tissues from WT and Lrrc19 KO mice 3 days after inoculation with UPEC strain CFT073 were analysed by qRT–PCR (upper). Transcriptional levels of TNFα, IL-6, MCP-1 and MIP-2 were shown as ‘fold increased’ relative to noninfection control. TNFα, IL-6, MCP-1 and MIP-2 in the sera of uninfected (uninf.) and UPEC-infected (Inf.) WT and Lrrc19 KO (L19KO) mice were analysed by ELISA (below). ( d ) Immunostaining analysis of cytokines in the kidney tissues from WT and Lrrc19 KO mice 3 days after inoculation with CFT073. Brown colour in immunostaining indicated positive response. Scale bars, 20 μm. * P <0.05 and ** P <0.01 ( t -test for two groups in c , mean±s.d. ; analysis of variance for multiple groups in c , mean±s.e.m., n =8 mice per group). The data are representative of at least three independent experiments. Full size image We next addressed whether LRRC19 could directly modulate the inflammatory responses of kidney tubular epithelial cells. The experiments were conducted using primary cultures of renal tubule epithelial cells microdissected from the kidneys of WT and Lrrc19 KO mice. These cells expressed cytokeratin 18 ( Fig. 3a ), consistent with other data [3] . Importantly, LRRC19 deficiency affected the phosphorylation of IκBα and degradation of IκBα in response to UPEC ( Fig. 3b and Supplementary Fig. 13 ). The nuclear translocation proportion of the transcriptional factor NF-κB p65, which is critical in the regulation of genes involved in inflammation [4] was also reduced in Lrrc19 KO renal tubular epithelial cells ( Fig. 3c ). LRRC19 also affected other inflammatory pathways. The phosphorylation of p38, Jun N-terminal kinase (JNK) and extracellular signal-regulated kinase (ERK), which are important for mediating inflammatory responses, was also significantly impaired in Lrrc19 KO renal tubular epithelial cells as compared with those in the WT kidney tubule cells in response to UPECs ( Fig. 3d and Supplementary Fig. 13 ). When UPEC were added into the culture, a dramatic increase in the expression of proinflammatory mediators, including TNF-α, IL-6, MCP-1 and MIP-2 was observed ( Supplementary Fig. 4 ). However, the levels of TNF-α, IL-6, MCP-1 and MIP-2 expression in Lrrc19 KO renal tubular epithelial cells were significantly lower than those in WT kidney tubular cells ( P <0.05, Fig. 3e ) in response to UPEC or its component LPS. Notably, the levels of TNF-α, IL-6, MCP-1 and MIP-2 expression in Lrrc19 KO renal tubular epithelial cells could be restored by transfecting plasmids encoding LRRC19 ( Fig. 3f and Supplementary Figs 5 and 17 ). Taken together, all of these indicate that LRRC19 indeed exerts a critical role in kidney against uropathogenic bacteria. Thus, LRRC19 expressed in renal tubule epithelial cells can modulate the inflammatory responses against UPEC. 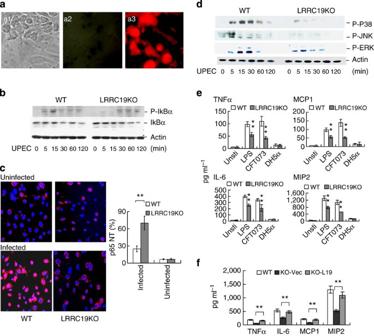Figure 3: LRRC19-deficient renal tubular epithelial cells have reduced inflammatory responses to UPEC. (a) Confluent culture of renal tubular epithelial cells. Murine renal tubular epithelial cells (a1) were identified by anti-cytokeratin antibody (a3). a2, isotypic control. Scale bars, 40 μm. (b) NF-κB activation analyses. The cells were lysed at the indicated time. Phosphor-IKBα or total IKBα was detected using anti-phosphor-IKBα or anti-IKBα antibody. (c) p65 nuclear translocation analysis. The rental tubular epithelial cells were stimulated withE. coliCFT073 (infected) or unstimulated (uninfected) for 3 h, then cells were stained with anti-p65 and Alexa Fluor 546–conjugated antibody, and then were counterstained for nucleic acids with DAPI (blue). Scale bar, 20 μm. NT, nuclear translocation. P65 NT(%)=cellular number with NT/total cellular number. A total of 1 × 103cells per sample were counted. (d) Phosphorylation analyses of p38, JNK and ERK. Murine kidney tubular cells from WT andLrrc19 KOmice were stimulated withE. coliCFT073. The cells were lysed at the indicated time. Phosphor-p38, -ERK and -JNK were detected using anti-phosphor-p38, -ERK or -JNK antibody. Actin, a loading control, was detected by anti-β-actin antibody. (e) ELISA analyses of TNFα, IL-6, MCP-1 and MIP-2. The cultured renal tubule epithelial cells were exposed to LPS,E. coliCFT073 or unpathogenic DH5αfor 24 h and then the supernatants were collected for ELISA. Unsti., negative control. (f) Functional restoration analyses ofLrrc19 KOrental tubular epithelial cells. The cultured renal tubule epithelial cells ofLrrc19 KOmice were transfected by vectors encoding LRRC19 or empty vectors. After transfection for 24 h, the cells were exposed toE. coliCFT073 for 24 h and then the supernatants were collected for ELISA. WT, the cultured renal tubular epithelial cells of WT mice; KO-Vec, LRRC19-deficient renal tubular epithelial cells transfected by empty vector; KO-L19, LRRC19-deficient renal tubular epithelial cells transfected by vector encoding LRRC19. *P<0.05 and **P<0.01 (t-test incandeand analysis of variance inf; mean±s.d.). The data are representative of three independent experiments. Figure 3: LRRC19-deficient renal tubular epithelial cells have reduced inflammatory responses to UPEC. ( a ) Confluent culture of renal tubular epithelial cells. Murine renal tubular epithelial cells (a1) were identified by anti-cytokeratin antibody (a3). a2, isotypic control. Scale bars, 40 μm. ( b ) NF-κB activation analyses. The cells were lysed at the indicated time. Phosphor-IKBα or total IKBα was detected using anti-phosphor-IKBα or anti-IKBα antibody. ( c ) p65 nuclear translocation analysis. The rental tubular epithelial cells were stimulated with E. coli CFT073 (infected) or unstimulated (uninfected) for 3 h, then cells were stained with anti-p65 and Alexa Fluor 546–conjugated antibody, and then were counterstained for nucleic acids with DAPI (blue). Scale bar, 20 μm. NT, nuclear translocation. P65 NT(%)=cellular number with NT/total cellular number. A total of 1 × 10 3 cells per sample were counted. ( d ) Phosphorylation analyses of p38, JNK and ERK. Murine kidney tubular cells from WT and Lrrc19 KO mice were stimulated with E. coli CFT073. The cells were lysed at the indicated time. Phosphor-p38, -ERK and -JNK were detected using anti-phosphor-p38, -ERK or -JNK antibody. Actin, a loading control, was detected by anti-β-actin antibody. ( e ) ELISA analyses of TNFα, IL-6, MCP-1 and MIP-2. The cultured renal tubule epithelial cells were exposed to LPS, E. coli CFT073 or unpathogenic DH5αfor 24 h and then the supernatants were collected for ELISA. Unsti., negative control. ( f ) Functional restoration analyses of Lrrc19 KO rental tubular epithelial cells. The cultured renal tubule epithelial cells of Lrrc19 KO mice were transfected by vectors encoding LRRC19 or empty vectors. After transfection for 24 h, the cells were exposed to E. coli CFT073 for 24 h and then the supernatants were collected for ELISA. WT, the cultured renal tubular epithelial cells of WT mice; KO-Vec, LRRC19-deficient renal tubular epithelial cells transfected by empty vector; KO-L19, LRRC19-deficient renal tubular epithelial cells transfected by vector encoding LRRC19. * P <0.05 and ** P <0.01 ( t -test in c and e and analysis of variance in f ; mean±s.d.). The data are representative of three independent experiments. Full size image LRRC19 promotes expression of antimicrobial substances Consistent with other data [6] , [7] , [8] , [9] , kidney also expressed different kinds of bactericidal substance ( Supplementary Fig. 6a ). Most of these bactericidal substances were higher in the UPEC-infected kidney tissue of WT mice than those in Lrrc19 KO mice ( Supplementary Fig. 6b ). As cathelicidin [21] , Reg3γ [22] and α-defensin-5 (ref. 23 ) have been supposed to have bactericidal function, we next further investigated their expression of in WT and Lrrc19 KO mice infected with UPEC. Reverse transcription–polymerase chain reaction (RT–PCR), western blot and immunostaining analyses showed that the levels of cathelicidins and Reg3γ expression were remarkably higher in the kidneys of UPEC-infected WT mice than in infected Lrrc19 KO mice ( P <0.05; Fig. 4a and Supplementary Figs 6b and 14 ). Enzyme-linked immunosorbent assay (ELISA) also revealed higher levels of α-defensin-5 in the kidney tissues of UPEC-infected WT mice than in those of Lrrc19 KO mice ( P <0.05; Fig. 4b ). We also examined the expression of cathelicidin, Reg3γ and α-defensin-5 by WT and Lrrc19 KO renal tubule epithelial cells in response to UPEC or its components in vitro . Similar to in vivo UPEC infection, Lrrc19 KO renal tubule epithelial cells had reduced expression of cathelicidin, Reg3γ and defensin-5 as compared with WT renal tubular epithelial cells ( Fig. 4c,d and Supplementary Fig. 14 ). Finally, we tested whether LRRC19 deficiency affected the bacteria-killing ability of kidney epithelial cells. Lrrc19 KO renal tubule epithelial cells indeed had the reduced ability to kill UPEC as compared with renal tubule epithelial cells from WT mice ( P <0.05; Fig. 4e ). Thus, deficiency of LRRC19 reduced expression of antimicrobial substance by kidney tissues in response to UPEC. 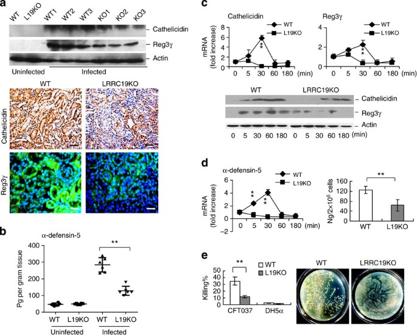Figure 4: LRRC19 deficiency reduces production of antimicrobial peptides and proteins by rental tubular epithelia cells in response to UPEC. (a) Immunoblot and immunostaining analyses of cathelicilin and Reg3γ in the uninfected and UPEC-infected kidneys of WT andLrrc19 KO(L19KO) mice. Brown colour indicated cathelicilin and green indicated Reg3γ (below). Scale bar, 40 μm. (b) ELISA analyses of α-defensin-5 in uninfected and infected kidney tissues WT andLrrc19 KO(L19KO) mice. Tissue was rinsed, homogenized and stored overnight at −20 °C. After two freeze–thaw cycles were performed to break the cell membranes, the homogenates were centrifuged and supernatants were removed, and α-defensin5 in the cellular lyses were detected by ELISA. (c) qRT–PCR and immunoblot analyses of cathelicilin and Reg3γ in the uninfected and UPEC-infected WT andLrrc19 KO(L19KO) kidney renal tubular epithelial cells. The cultured renal tubular epithelial cells were exposed toE. coliCFT073 and total RNAs were extracted at the indicated time. The relative fold increase of each mRNA levels compared with the PBS control group was reported as means±s.d. from duplicate measurements. The proteins of cathelicilin and Reg3γ in the cellular lysis were detected by immunoblot. (d) qRT–PCR and ELISA analyses of α-defensin-5 in the uninfected and UPEC-infected WT andLrrc19 KO(L19KO) kidney renal tubular epithelial cells. The cultured renal tubular epithelial cells were exposed toE. coliCFT073 and total RNAs were extracted and supernatants were collected at the indicated time. (e) Bactericidal analyses by WT andLrrc19 KOrenal epithelial cells on UPEC. Renal tubular epithelial cells from WT andLrrc19 KOmice were stimulated by heat-killed CFT073 or DH5 α for 18 h and then supernatants were collected for bactericidal analyses. *P<0.05 and **P<0.01 (Mann–WhitneyUtest inb;t-test, mean±s.d. inc,dande). The data are representative of three independent experiments. Figure 4: LRRC19 deficiency reduces production of antimicrobial peptides and proteins by rental tubular epithelia cells in response to UPEC. ( a ) Immunoblot and immunostaining analyses of cathelicilin and Reg3γ in the uninfected and UPEC-infected kidneys of WT and Lrrc19 KO (L19KO) mice. Brown colour indicated cathelicilin and green indicated Reg3γ (below). Scale bar, 40 μm. ( b ) ELISA analyses of α-defensin-5 in uninfected and infected kidney tissues WT and Lrrc19 KO (L19KO) mice. Tissue was rinsed, homogenized and stored overnight at −20 °C. After two freeze–thaw cycles were performed to break the cell membranes, the homogenates were centrifuged and supernatants were removed, and α-defensin5 in the cellular lyses were detected by ELISA. ( c ) qRT–PCR and immunoblot analyses of cathelicilin and Reg3γ in the uninfected and UPEC-infected WT and Lrrc19 KO (L19KO) kidney renal tubular epithelial cells. The cultured renal tubular epithelial cells were exposed to E. coli CFT073 and total RNAs were extracted at the indicated time. The relative fold increase of each mRNA levels compared with the PBS control group was reported as means±s.d. from duplicate measurements. The proteins of cathelicilin and Reg3γ in the cellular lysis were detected by immunoblot. ( d ) qRT–PCR and ELISA analyses of α-defensin-5 in the uninfected and UPEC-infected WT and Lrrc19 KO (L19KO) kidney renal tubular epithelial cells. The cultured renal tubular epithelial cells were exposed to E. coli CFT073 and total RNAs were extracted and supernatants were collected at the indicated time. ( e ) Bactericidal analyses by WT and Lrrc19 KO renal epithelial cells on UPEC. Renal tubular epithelial cells from WT and Lrrc19 KO mice were stimulated by heat-killed CFT073 or DH5 α for 18 h and then supernatants were collected for bactericidal analyses. * P <0.05 and ** P <0.01 (Mann–Whitney U test in b ; t -test, mean±s.d. in c , d and e ). The data are representative of three independent experiments. Full size image LRRC19-induced inflammation is through TRAF2 and TRAF6 As LRRC19 can bind to TLR ligands ( Supplementary Fig. 7b ) in LRRC19 stably transfected HEK293T cells and initiate innate immune responses in the similar way as do other TLRs do [24] , we suggested that there might be some overlap between LRRC19 and TLR-mediated signalling pathways. To test this hypothesis, we employed a knockdown technique to examine the potential adaptive molecules that may be involved in LRRC19-mediated activation using LRRC19 expressing HEK293T cells, which do not express endogenous TLRs but do have fully functional TLR signalling machinery [25] . We found that silencing TRAF2, TRAF6, TAK1-binding protein 2 (TAB2), TAK1-binding protein 3 (TAB3) or p65 but not MyD88, TRIF, IRAK1 and IRAK4 affected the LRRC19-mediated inflammatory cytokine IL-8 production or NF-κB activation in response to TLR4 ligand LPS or TLR1/2 ligand PAM3CSK4 ( Fig. 5a and Supplementary Fig. 7d ). In contrast, LPS or PAM3CSK4-mediated inflammatory responses in TLR4 or TLR1/2 expressing HEK293T cells were affected not only by siRNAs targeting TRAF2, TRAF6, TAB2, TAB3 or p65 but also by siRNAs targeting MyD88, TRIF, IRAK1 and IRAK4 ( Fig. 5a and Supplementary Fig. 7d ). The transfection of TRAF2, TRAF6 or TRAF2/6 also promoted the LRRC19-mediated IL-8 production in LRRC19 expressing HEK293T cells ( Supplementary Fig. 8b ). These findings suggest that LRRC19-mediated activation may be independent of MyD88, which have a critical role in TLRs such as TLR4- and TLR1/2-mediated inflammatory responses. To further confirm this finding, we performed silencing and overexpressing experiments of MyD88 in WT, Lrrc19 KO and Tlr4 KO renal tubule epithelial cells, the expression of inflammatory factor MIP-2 could be affected by silencing or overexpressing MyD88 in WT, LRRC19 KO but not in Tlr4 KO renal tubule epithelial cells in response to LPS ( Supplementary Fig. 8c,d ). Thus, LRRC19-mediated activation may directly be through TRAF2 and TRAF6 adaptive molecules, which have a critical role in NF-κB and MAPK signal pathways. 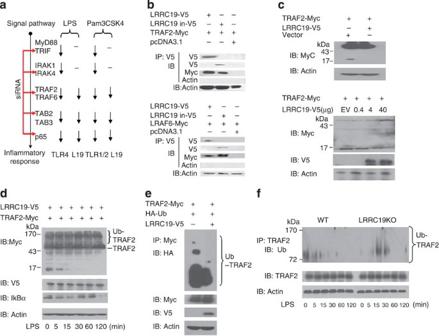Figure 5: LRRC19 inhibits the degradation of TRAF2. (a) Schematic diagram showing adaptive molecules which are involved in LRRC19-induced activation, based on data inSupplementary Fig. 6; ‘↓’ indicates reduced inflammatory responses, whereas ‘—’ indicates no effect after exposure to LPS or Pam3CSK4 while the adaptive molecules in TLR-MyD88 signal pathway were silenced. (b) Immunoblot assay in HEK293T cells transfected to express TRAF2-Myc (upper) or TRAF6-Myc (below) with or without V5-tagged LRRC19 (LRRC19-V5) or V5-tagged LRRC19 intracellular domain (LRRC19-in-V5). Immunoprecipitation was performed by anti-V5 agarose. LRRC19 or LRRC19 intracellular domain and TRAF2 or TRAF6 were analysed by detecting V5 or myc using antibody specific for V5 and myc. (c) Immunoblot assay of TRAF2 in TRAF2 and LRRC19-co-transfected HEK293T cells. HEK293T cells were transfected by Myc-tagged TRAF2 (TRAF2-Myc) with (+) or without (-) V5-tagged LRRC19 (LRRC19-V5). The expression of TRAF2 and LRRC19 were analysed by detecting myc and V5 expression using antibody specific for myc and V5 after transfection for 24 h. The degradated fragment (17 kDa fragment) from TRAF2 was shown in the blots. Vector or EV, control empty vector. (d) Immunoblot assay of TRAF2 in LRRC19 and TRAF2 co-expressing HEK293T cells. HEK293T cells were transfected by Myc-tagged TRAF2 (TRAF2-Myc) with V5-tagged LRRC19 (LRRC19-V5, 0.4 μg) and then stimulated by LPS. The degradated fragment (17 kDa) and ubiquitinated TRAF2 (Ub-TRAF2) were analysed using antibody specific for myc (upper blots) at the indicated time. LRRC19, IκBα and actin were also analysed using antibody specific for V5, IκBα or actin in the same cells (below blots). (e) Immunoblot analysis of the ubiquitination of TRAF2 in HEK293T cells transfected to express Myc-tagged TRAF2 (TRAF2-Myc) and hemagglutinin-tagged ubiquitin (HA-Ub) in the presence (+) or absence (−) of vector encoding V5-tagged LRRC19, assessed after (top) or without (below) immunoprecipitation with anti-myc agarose. (f) Immunoblot analysis of ubiqitinated TRAF2 and TRAF2 immunoprecipitated from WT andLrrc19 KOrental tubular epithelial cells stimulated with LPS at the indicated time (upper blots), and actin (below blot) in the same cells without immunoprecipitation. IB, immunoblot assay; IP, immunoprecipitation. Figure 5: LRRC19 inhibits the degradation of TRAF2. ( a ) Schematic diagram showing adaptive molecules which are involved in LRRC19-induced activation, based on data in Supplementary Fig. 6 ; ‘↓’ indicates reduced inflammatory responses, whereas ‘—’ indicates no effect after exposure to LPS or Pam3CSK4 while the adaptive molecules in TLR-MyD88 signal pathway were silenced. ( b ) Immunoblot assay in HEK293T cells transfected to express TRAF2-Myc (upper) or TRAF6-Myc (below) with or without V5-tagged LRRC19 (LRRC19-V5) or V5-tagged LRRC19 intracellular domain (LRRC19-in-V5). Immunoprecipitation was performed by anti-V5 agarose. LRRC19 or LRRC19 intracellular domain and TRAF2 or TRAF6 were analysed by detecting V5 or myc using antibody specific for V5 and myc. ( c ) Immunoblot assay of TRAF2 in TRAF2 and LRRC19-co-transfected HEK293T cells. HEK293T cells were transfected by Myc-tagged TRAF2 (TRAF2-Myc) with (+) or without (-) V5-tagged LRRC19 (LRRC19-V5). The expression of TRAF2 and LRRC19 were analysed by detecting myc and V5 expression using antibody specific for myc and V5 after transfection for 24 h. The degradated fragment (17 kDa fragment) from TRAF2 was shown in the blots. Vector or EV, control empty vector. ( d ) Immunoblot assay of TRAF2 in LRRC19 and TRAF2 co-expressing HEK293T cells. HEK293T cells were transfected by Myc-tagged TRAF2 (TRAF2-Myc) with V5-tagged LRRC19 (LRRC19-V5, 0.4 μg) and then stimulated by LPS. The degradated fragment (17 kDa) and ubiquitinated TRAF2 (Ub-TRAF2) were analysed using antibody specific for myc (upper blots) at the indicated time. LRRC19, IκBα and actin were also analysed using antibody specific for V5, IκBα or actin in the same cells (below blots). ( e ) Immunoblot analysis of the ubiquitination of TRAF2 in HEK293T cells transfected to express Myc-tagged TRAF2 (TRAF2-Myc) and hemagglutinin-tagged ubiquitin (HA-Ub) in the presence (+) or absence (−) of vector encoding V5-tagged LRRC19, assessed after (top) or without (below) immunoprecipitation with anti-myc agarose. ( f ) Immunoblot analysis of ubiqitinated TRAF2 and TRAF2 immunoprecipitated from WT and Lrrc19 KO rental tubular epithelial cells stimulated with LPS at the indicated time (upper blots), and actin (below blot) in the same cells without immunoprecipitation. IB, immunoblot assay; IP, immunoprecipitation. Full size image We next addressed how LRRC19 induce inflammatory responses through TRAF2 and TRAF6. Immunoprecipitation analyses showed the binding of LRRC19 intracellular region with TRAF2 and TRAF6 ( Fig. 5b ). Meanwhile, confocal observation also revealed the colocalization of LRRC19 and TRAF2 or TRAF6 ( Supplementary Fig. 8a ) in LRRC19 and TRAF2 or TRAF6 co-expressing HEK293T cells. As TRAF6 and TRAF2 could be ubiquitinated in the process of signal transduction [26] , [27] , [28] , we hypothesized that the interaction of LRRC19 and TRAF6 or TRAF2 could affect the ubiquitination of TRAF6 and TRAF2. While the cells were transfected using Myc-tagged TRAF2 with control empty plasmid, degradation of TRAF2 could be observed ( Fig. 5c ). However, this degradation could be inhibited by LRRC19 in HEK293T cells co-expressing V5-tagged LRRC19 and Myc-tagged TRAF2; furthermore, strengthened inhibition could be observed with increased LRRC19 ( Fig. 5c and Supplementary Fig. 15 ). To further determine the effect of LRRC19 on TRAF2 degradation upon the exposure to UPEC, we co-transfected HEK293T cells using lower dose of LRRC19 with TRAF2. We found that LRRC19-mediated inhibition could be further strengthened by LPS ( Fig. 5d and Supplementary Fig. 15 ). Similar phenomenon was not found in HEK293T cells co-expressing LRRC19 and TLR4 ( Supplementary Figs 9 and 17 ), further suggesting that LRRC19-mediated inflammatory responses is independent of TLR4-MyD88-mediated signalling. To explain LRRC19-mediated suppression on TRAF2 degradation, we next investigated the effects of LRRC19 on the ubiquitination of TRAF2 molecules. We transfected HEK293T cells to express Myc-tagged TRAF2, as well as hemagglutinin-tagged ubiquitin in the presence or absence of V5-tagged LRRC19. The presence of LRRC19 indeed resulted in less uniquitination of TRAF2 ( Fig. 5e and Supplementary Fig. 15 ). We also transfected WT kidney epithelial cells to overexpress LRRC19. The uniquitination of TRAF2 could be suppressed in the LRRC19 overexpressing kidney epithelial cells ( Supplementary Figs 10 and 17 ). The ubiquitination of TRAF2 was also remarkably inhibited in WT renal tubular epithelial cells; whereas the ubiquitination in Lrrc19 KO was remarkably promoted in response to LPS ( Fig. 5f and Supplementary Fig. 15 ). As TRAF2 have an important role in mediating inflammatory response, when renal tubular epithelial cells were exposed to UPEC, LRRC19 could inhibit the degradation of TRAF2 through decreasing uniquitination of TRAF2 to promote inflammatory responses. We next investigated the effect of LRRC19 on the TRAF6. While HEK293T cells were co-transfected by V5-tagged LRRC19 with Myc-tagged TRAF6, the levels of TRAF6 proteins decreased with the increased dose of LRRC19 ( Fig. 6a and Supplementary Fig. 16 ) and was remarkably ubiquitinated in response to LPS ( Fig. 6b and Supplementary Fig. 16 ). Notably, LRRC19-mediated ubiquitination of TRAF6 is completely different from TLR4 ( Fig. 6b ), again indicating that LRRC19 is independent of TLR4-MyD88 to mediate inflammatory responses. To further determine the effects of LRRC19 on the ubiquitination of TRAF6 molecules, we transfected HEK293T cells to express Myc-tagged TRAF6, as well as hemagglutinin-tagged ubiquitin in the presence or absence of V5-tagged LRRC19. The presence of LRRC19 indeed resulted in more uniquitination of TRAF6 ( Fig. 6c and Supplementary Fig. 16 ). Although proteins are frequently targeted to the proteosome for degradation by conjugation with K48-linked ubiquitin chains, K63-linked ubiquitin is a common activating signal [29] , [30] . Thus, to determine the type of ubiquitin on TRAF6 that was affected by LRRC19, we transfected HEK293T cells to express TRAF6 with LRRC19 in the presence of vector encoding total ubiquitin, K48-linked ubiquitin or K63-linked ubiquitin. LRRC19 resulted in more total ubiquitin on TRAF6, accompanied by more K63-linked ubiquitin ( Fig. 6d and Supplementary Fig. 16 ). We also immunoprecipitated endogenous TRAF6 and measured K63 or K48-linked ubiquitin associated with TRAF6 by timed stimulation. There was remarkable K63-linked ubiquitin on TRAF6 from WT; whereas K63-linked ubiquitin was hard to be detected on TRAF6 from Lrrc19 KO renal tubular epithelial cells ( Fig. 6e and Supplementary Fig. 16 ). Thus, these data demonstrate that LRRC19 may mediate K63-linked ubiquitination of TARF6, which can promote downstream signalling [31] . Notably, the inhibition of K48-linked ubiquitination of TRAF6 was observed in the presence of LRRC19 ( Supplementary Figs 11 and 17 ), however, the presence of LRRC19 indeed caused decrease and uniquitination of TRAF6 ( Fig. 6a,c ), indicating that the inhibition of K48-linked ubiquitination of TRAF6 does not impede the other ubiquitin-mediated degradation of TRAF6. Taken together, these results suggest that LRRC19-induced innate immune responses against UPEC infection are mediated not only through inhibiting degradation of TRAF2 but also increasing K63-linked ubiquitin on TRAF6 (s). 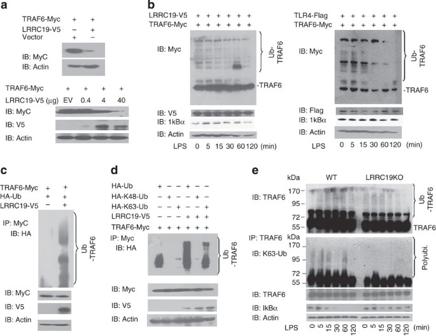Figure 6: LRRC19 promotes K63-linked ubiquitination of TRAF6. (a) Immunoblot assay of TRAF6 in TRAF6 and LRRC19 co-expressing HEK293T cells. HEK293T cells were transfected by Myc-tagged TRAF6 (TRAF6-Myc) with (+) or without (−) V5-tagged LRRC19 (LRRC19-V5) (upper) or different doses of LRRC19-V5 (below). The expression of TRAF6 and LRRC19 were analysed by detecting myc and V5 expression using antibody specific for myc and V5 after transfection for 24 h. Vector or EV, control empty vector. (b) Immunoblot assay of TRAF6 in TRAF6 and LRRC19 or TLR4 co-expressing HEK293T cells. HEK293T cells were transfected by Myc-tagged TRAF6 (TRAF6-Myc) with V5-tagged LRRC19 (LRRC19-V5; right) or Flag-tagged TLR4 (TLR4-Flag; left) and then stimulated by LPS. The ubiquitinated TRAF6 (Ub-TRAF6), LRRC19 and TLR4 were analysed by detecting myc, V5 or flag expression using antibody specific for myc, V5 and flag at the indicated time. IκBα and actin from the same cells were also detected by specific antibodies. (c) Immunoblot analysis of the ubiquitination of TRAF6 in HEK293T cells transfected to express Myc-tagged TRAF6 (TRAF6-Myc) and hemagglutinin-tagged ubiquitin (HA-Ub) in the presence (+) or absence (−) of vector encoding V5-tagged LRRC19, assessed after (top) or without (below) immunoprecipitation with anti-myc agarose. (d) Immunoblot analysis of K48-linked and K63-linked ubiquitination of TRAF6 in the cells transfected to express Myc-TRAF6 (TRAF6-Myc) with or without V5-tagged LRRC19 (LRRC19-V5), plus vectors encoding hemagglutinin-tagged total ubiquitin (HA-Ub), K48-linked ubiquitin (HA-48-Ub) or K63-linked ubiquitin (HA-K63-Ub) and immunoblot analysis of TRAF6 (myc), LRRC19 (V5) and actin (below blots) in the same cells without immunoprecipitation. (e) Immunoblot analysis of K63-linked ubiquitination (K63-Ub) of endogenouse TRAF6 immunoprecipitated from WT andLrrc19 KOrental tubular epithelial cells stimulated with LPS (middle blot), and immunoblot analysis of Ub-TRAF6 (top blot), TRAF6, IkBα and actin (below blots) in the same cells without immunoprecipitation. IB, immunoblot assay; IP, immunoprecipitation; PolyUbi., polyubiquitination. Figure 6: LRRC19 promotes K63-linked ubiquitination of TRAF6. ( a ) Immunoblot assay of TRAF6 in TRAF6 and LRRC19 co-expressing HEK293T cells. HEK293T cells were transfected by Myc-tagged TRAF6 (TRAF6-Myc) with (+) or without (−) V5-tagged LRRC19 (LRRC19-V5) (upper) or different doses of LRRC19-V5 (below). The expression of TRAF6 and LRRC19 were analysed by detecting myc and V5 expression using antibody specific for myc and V5 after transfection for 24 h. Vector or EV, control empty vector. ( b ) Immunoblot assay of TRAF6 in TRAF6 and LRRC19 or TLR4 co-expressing HEK293T cells. HEK293T cells were transfected by Myc-tagged TRAF6 (TRAF6-Myc) with V5-tagged LRRC19 (LRRC19-V5; right) or Flag-tagged TLR4 (TLR4-Flag; left) and then stimulated by LPS. The ubiquitinated TRAF6 (Ub-TRAF6), LRRC19 and TLR4 were analysed by detecting myc, V5 or flag expression using antibody specific for myc, V5 and flag at the indicated time. IκBα and actin from the same cells were also detected by specific antibodies. ( c ) Immunoblot analysis of the ubiquitination of TRAF6 in HEK293T cells transfected to express Myc-tagged TRAF6 (TRAF6-Myc) and hemagglutinin-tagged ubiquitin (HA-Ub) in the presence (+) or absence (−) of vector encoding V5-tagged LRRC19, assessed after (top) or without (below) immunoprecipitation with anti-myc agarose. ( d ) Immunoblot analysis of K48-linked and K63-linked ubiquitination of TRAF6 in the cells transfected to express Myc-TRAF6 (TRAF6-Myc) with or without V5-tagged LRRC19 (LRRC19-V5), plus vectors encoding hemagglutinin-tagged total ubiquitin (HA-Ub), K48-linked ubiquitin (HA-48-Ub) or K63-linked ubiquitin (HA-K63-Ub) and immunoblot analysis of TRAF6 (myc), LRRC19 (V5) and actin (below blots) in the same cells without immunoprecipitation. ( e ) Immunoblot analysis of K63-linked ubiquitination (K63-Ub) of endogenouse TRAF6 immunoprecipitated from WT and Lrrc19 KO rental tubular epithelial cells stimulated with LPS (middle blot), and immunoblot analysis of Ub-TRAF6 (top blot), TRAF6, IkBα and actin (below blots) in the same cells without immunoprecipitation. IB, immunoblot assay; IP, immunoprecipitation; PolyUbi., polyubiquitination. Full size image LRRC19 is a main contributor to renal infection defense We finally compared the contribution of LRRC19 and other pathogen-recognition receptors in preventing infection by UPEC in kidney. Previous data indicate that TLR4 (ref. 32 ), TLR5 (ref. 5 ) and TLR11 (ref. 16 ) have a role in eliminating UPEC by the kidney. However, TLR5 mainly exerts its role in bladder where TLR5 is highly expressed [5] and TLR11 is not expressed in human kidney [16] . Therefore, we only compared the contribution of LRRC19 and TLR4 in preventing infection by UPEC in kidney. When Lrrc19 KO , Tlr4 KO mice and control MyD88 KO mice were transurethrally inoculated with 5.0 × 10 7 CFUs of UPEC CFT073, Lrrc19 KO mice had a median of 1 × 10 3 CFU per gram kidney tissue; whereas Tlr4 KO mice had a median of 4.5 × 10 2 CFU per gram tissue ( P <0.01) at 3 days post inoculation ( Fig. 7a ). Furthermore, a median of CFU per gram kidney tissue was still higher in Tlr4 KO mice than those in Lrrc19 KO mice at 7 days post infection ( Fig. 7a ), suggesting LRRC19 may exert a more important role in eliminating UPEC in the kidney tissues. In addition, there was a weaker inflammatory response in Lrrc19 KO mice than Tlr4 KO mice, such as the lower levels of TNFα, IL-6, MCP-1 and MIP-2 and fewer inflammatory cells in the spleens of infected Lrrc19 KO mice ( Fig. 7b–d and Supplementary Fig. 12 ). The bladders of the infected Lrrc19 KO mice, unlike the Tlr4 KO and MyD88 KO mice, had less CFUs with strong inflammation, including prominent submucosal oedema and leukocyte infiltration of the submucosa and epithelium ( Fig. 7 and Supplementary Fig. 12 ). This may be derived from the fact that LRRC19 does not express in the bladder ( Fig. 1 ). Thus, these data indicate that LRRC19 may be a main defender against UPEC in the kidney. 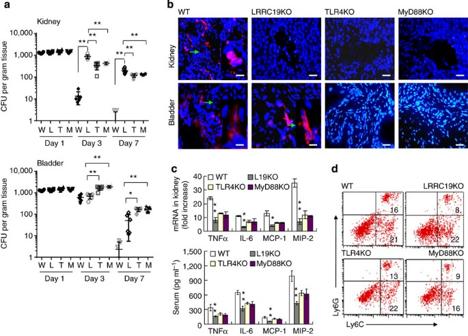Figure 7: LRRC19 is a main contributor in preventing infection by UPEC in the kidney. (a) Bacterial counts in the kidney (upper) and bladder (below) of UPEC-infected WT (W),Lrrc19 KO(L),Tlr4 KO(T) andMyD88 KO(M) mice. Mice were inoculated transurethrally with 5.0 × 107E. coliCFT073. Then 1, 3 and 7 days post infection, kidney and bladder were removed from infected mice and the homogenates were plated on LB agar to enumerate CFU per gram tissue. Colony counts are the mean of three plates per mouse. (b) Immunostaining observation of the kidney and bladder from UPEC-infected WT,Lrrc19 KO,Tlr4 KOandMyd88 KOmice. 5-μm-thick sections of the kidney or bladder from the UPEC-infected WT,Lrrc19 KO,Tlr4 KOorMyd88 KOmice, which were prepared from frozen tissue, were stained by PE-labelled anti-Ly6G antibody (red) and DAPI (blue). Arrow, neutrophils. Scale bars, 20 μm. (c) qRT–PCR and ELISA analyses of TNFα, IL-6, MCP-1 and MIP-2. Expression of proinflamamtory mediators was analysed by qRT–PCR in kidneys from WT, Lrrc19 KO,Tlr4 KO, andMyD88 KOmice 3 days after inoculation with UPEC strain CFT073 (upper). Results are shown as ‘fold increased’ relative to noninfection control. TNFα, IL-6, MCP-1 and MIP-2 in the sera of UPEC-infected WT, Lrrc19 KO,Tlr4 KOandMyD88 KOmice 3 days after inoculation with UPEC strain CFT073 were analysed using ELISA kits (below). (d) Flow cytometry analysis of inflammatory cells. Splenocytes of UPEC- infected WT,Lrrc19 KO,Tlr4 KOandMyD88 KOmice were stained by anti-Ly6G and Ly6C and then analysed by FACScan. Numbers indicate percentage of Ly6G+Ly6C+or Ly6C+cells. *P<0.05 and **P<0.01 (Mann–WhitneyUtest ina; analysis of variance test inc, mean±s.e.m.,n=8 mice per group). The data were representative of three independent experiments. Figure 7: LRRC19 is a main contributor in preventing infection by UPEC in the kidney. ( a ) Bacterial counts in the kidney (upper) and bladder (below) of UPEC-infected WT (W), Lrrc19 KO (L), Tlr4 KO (T) and MyD88 KO (M) mice. Mice were inoculated transurethrally with 5.0 × 10 7 E. coli CFT073. Then 1, 3 and 7 days post infection, kidney and bladder were removed from infected mice and the homogenates were plated on LB agar to enumerate CFU per gram tissue. Colony counts are the mean of three plates per mouse. ( b ) Immunostaining observation of the kidney and bladder from UPEC-infected WT, Lrrc19 KO , Tlr4 KO and Myd88 KO mice. 5-μm-thick sections of the kidney or bladder from the UPEC-infected WT, Lrrc19 KO , Tlr4 KO or Myd88 KO mice, which were prepared from frozen tissue, were stained by PE-labelled anti-Ly6G antibody (red) and DAPI (blue). Arrow, neutrophils. Scale bars, 20 μm. ( c ) qRT–PCR and ELISA analyses of TNFα, IL-6, MCP-1 and MIP-2. Expression of proinflamamtory mediators was analysed by qRT–PCR in kidneys from WT , Lrrc19 KO , Tlr4 KO , and MyD88 KO mice 3 days after inoculation with UPEC strain CFT073 (upper). Results are shown as ‘fold increased’ relative to noninfection control. TNFα, IL-6, MCP-1 and MIP-2 in the sera of UPEC-infected WT , Lrrc19 KO , Tlr4 KO and MyD88 KO mice 3 days after inoculation with UPEC strain CFT073 were analysed using ELISA kits (below). ( d ) Flow cytometry analysis of inflammatory cells. Splenocytes of UPEC- infected WT, Lrrc19 KO , Tlr4 KO and MyD88 KO mice were stained by anti-Ly6G and Ly6C and then analysed by FACScan. Numbers indicate percentage of Ly6G + Ly6C + or Ly6C + cells. * P <0.05 and ** P <0.01 (Mann–Whitney U test in a ; analysis of variance test in c , mean±s.e.m., n =8 mice per group). The data were representative of three independent experiments. Full size image In this study, we demonstrate that Lrrc19 KO mice are more susceptible than WT and even Tlr4 KO mice to UPEC infection. We found that LRRC19 in renal tubular epithelial cells not only modulates the expression of inflammatory cytokines and chemokines, but also antimicrobial peptides and proteins. Finally, we identify LRRC19-mediated signal pathway in which LRRC19 may mediate more K63-linked ubiquitin on TRAF6 and inhibit the degradation of TRAF2 through direct interaction with TRAF6 or TRAF2 to activate NF-κB and MAPK pathways. Meanwhile, our results suggest a cooperative network constructed by LRRC19, TLR4 and TNF-α-mediated signalling pathways to effectively prevent and eliminate UPEC infection in kidney tissues ( Fig. 8 ). 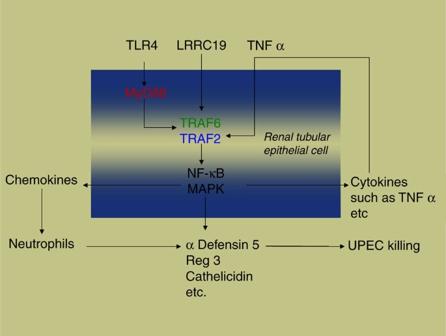Figure 8: Signalling network induced to prevent and eliminate UPEC infection in kidney tissues. In response to UPEC infection, the bacteria activate NF-κB and MAPK not only through the TLR4-mediated MyD88 signalling pathway but also through LRRC19-mediated TRAF2 and TRAF6 signalling pathways. As TRAF6 is a common molecule of the TLR4-MyD88-TRAF6 and LRRC19-TRAF6 pathways, there may be a cooperative effect on the activation of NF-κB and MAPK. TRAF2 also mediates the signal transduction from members of the TNF receptor superfamily34,35, such as TNFα, which can be produced by kidney tubular epithelial cells so that there may be cooperation between the LRRC19 and TNFα-mediated signals. Thus, there may exist a cooperative network constructed by LRRC19, TLR4 and TNFα-mediated signalling pathways in the kidney against UPEC. Figure 8: Signalling network induced to prevent and eliminate UPEC infection in kidney tissues. In response to UPEC infection, the bacteria activate NF-κB and MAPK not only through the TLR4-mediated MyD88 signalling pathway but also through LRRC19-mediated TRAF2 and TRAF6 signalling pathways. As TRAF6 is a common molecule of the TLR4-MyD88-TRAF6 and LRRC19-TRAF6 pathways, there may be a cooperative effect on the activation of NF-κB and MAPK. TRAF2 also mediates the signal transduction from members of the TNF receptor superfamily [34] , [35] , such as TNFα, which can be produced by kidney tubular epithelial cells so that there may be cooperation between the LRRC19 and TNFα-mediated signals. Thus, there may exist a cooperative network constructed by LRRC19, TLR4 and TNFα-mediated signalling pathways in the kidney against UPEC. Full size image Multiple members of the LRR protein family, including LRRC19 and TLRs, are involved in the clearance of UPEC from kidney tissues. Renal tubular epithelial cells express multiple TLRs such as TLR1, 2, 3, 4, 6 and 11 (ref. 12 ), which contribute to the host innate immune responses to UTI by UPEC. Others have found that deficiency of TLR2 (ref. 15 ), TLR4 (ref. 14 ), TLR5 (ref. 5 ) and TLR11 (ref. 16 ) increases susceptibility to UTIs. Our results demonstrate that LRRC19 deficiency impairs the ability of the kidney to eliminate UPEC accompanied by reduced inflammatory responses. Furthermore, we also found that LRRC19 in renal epithelial cells has a more important role even than TLR4 in host defense against Gram-negative UPEC in the kidney. LRRC19 is a member of the LRR_only protein group [11] and differs from TLRs in that it does not have a TIR domain. Notably, while the negative impact of the impaired inflammatory responses in Lrrc19 KO mice are present, detrimental effects associated to inflammation in WT mice may potentially damage kidney function. Anyway, LRRC19 expressed in kidney tubular epithelial cells recognize microbial pathogens and induce inflammatory responses by activating NF-κB and MAPK signalling pathways. Our results suggest a cooperative network constructed by LRRC19, TLR4 and TNF-α-mediated signalling pathways. Previous studies have implied that different bacterial factors produced by UPEC may be implicated in the activation of both TLR4-dependent and -independent signalling pathways [3] . We here demonstrate the critical roles of LRRC19 in TLR4-MyD88-independent signalling pathways. In response to UPEC infection, LRRC19 may activate NF-κB and MAPK through directly interacting with TRAF2 and TRAF6 signalling pathways. This is consistent with the critical role of TRAF2 and TRAF6 in TLR4-independent signalling pathways [3] . Thus, in the cases of UTI, the bacteria activate NF-κB and MAPK not only through the TLR4-mediated MyD88 signalling pathway but also through LRRC19-mediated TRAF2 and TRAF6 signalling pathways. As TRAF6 is a common molecule of the TLR4-MyD88-TRAF6 and LRRC19-TRAF6 pathways, there may be a cooperative effect on the activation of NF-κB and MAPK. LRRC19, which promotes the production of inflammatory cytokines in vivo and improved health in UPEC. Furthermore, our study has provided a mechanism whereby LRRC19 positively affected LPS signalling by associating with TRAF6, which led to several effects on TRAF6, including more K63-linked ubiquitination of TRAF6, followed by more activation and nuclear translocation NF-κB. Several approaches show that ubiquitination and proteasomal activity are integral to TRAF2 degradation, and inhibition of this process potentiates signalling [33] . Our data exhibit the interaction of LRRC19 with TRAF2 to inhibit the degradation of TRAF2. Since TRAF2 mediates the signal transduction from members of the TNF receptor superfamily [34] , [35] such as TNFα, which can be produced by kidney tubular epithelial cells, thus there may exist cooperation between the LRRC19 and TNFα-mediated signals also. In addition, TRAF6 may interact with various protein kinases including interleukin1 receptor-associated kinase (IRAK1/IRAK) [36] , SRC and protein kinase C (PKC) ζ [37] , which provide a link between distinct signalling pathways. TRAF6 protein may also interact with UBE2N/UBC13 (ref. 38 ) and UBE2V1/UEV1A [39] , which is required for IκB kinase (IKK) activation. Thus, there may be a network constructed of LRRC19, TLR4 and TNF-α-mediated signalling pathway (s) to effectively prevent and eliminate UPEC infection in kidney tissue. Renal epithelial cells can produce cytokines, chemokines and antimicrobial peptides following bacterial stimulation [40] . Chimeric mice generated by infusing Lrrc19 KO BM cells into lethally irradiated WT recipient mice demonstrate the important roles of LRRC19 in kidney tubular epithelial cells-mediated inflammatory responses. Patole et al . [41] have also reported that TLR4 is required not only by BM-derived cells but also by intrinsic renal tubule cells to initiate chemokine-derived, renal neutrophil recruitment. Moreover, LRRC19 expressed in kidney tubular cells not only modulated the expression of inflammatory cytokines but also antimicrobial peptides and proteins, such as α-defensin-5, Reg3γ and cathelicidin. Importantly, we found that LRRC19-deficient kidney tubular cells also have a reduced ability to kill UPEC, consistent with the fact that the antimicrobial substances have antibacterial activity against common uropathogenic Gram-positive bacteria and Gram-negative bacteria [6] , [8] , [9] , [10] . Thus, LRRC19 in kidney tubule cells is involved not only in attracting inflammatory cells but also in kidney-mediated killing of uropathogenic bacteria. In summary, the present study helps to elucidate the role of LRRC19 in preventing UTI, and provides evidence that LRRC19 mediates the production of cytokines, chemokines and antimicrobial peptides and proteins through TRAF2 and TRAF6 signalling pathways. To our knowledge, LRRC19 represents the first identified LRR-containing molecule capable of activating NF-κB and MAPK via direct interaction with TRAF2 and TRAF6 in the kidney tubular epithelial cells. Our findings provide new insight into the understanding of inflammatory responses, which will have important consequences for developing new strategies against UPEC infection. Lrrc19 KO mice Bacterial artificial chromosome (BAC)-retrieval was used to construct the targeting vector. In brief, the LRRC19 gene was acquired from a C57BL/6J BAC clone (RP24-370N3, provided by the BACPAC Resource Center) using a vector containing two homologous arms. After correct recombination, this vector contains 15.5 kb of genomic sequence including part of intron I, exons II–V and 4.1 kb of downstream sequence. To construct a targeting vector, the entire region encompassing exons II–IV and 304 bp of exon V of Lrrc19 was then replaced with a loxP-neomycin resistance (neo)-loxP cassette. The neo cassette was in the reverse transcriptional orientation compared with the Lrrc19 . The targeting construct which contains a neo cassette for positive selection and a herpes simplex virus-thymidine kinase expression cassette for negative selection was linearized with Not I and electroporated into C57BL/6-derived B6/BLU embryonic stem (ES) cells. Ninety-six ES cell clones were selected and examined for correct recombination using long-range PCR and Southern blot analysis. Probes for Southern blot analysis were listed in Supplementary Table 1(a) . Correctly-targeted ES cells were injected into C57BL/6J blastocysts followed by transfer to pseudopregnant mice. Chimeric male mice identified by PCR were bred with C57BL/6J females to generate F1 offspring. Germline transmission of the targeted LRRC19 allele was verified by PCR analysis of DNA exacted from tails of F1 offspring. All the procedures were conducted according to the Institutional Animal Care and Use Committee of the Model Animal Research Center. Primers used in this experiment were listed in Supplementary Table 1(b) . Chimeric mice Six-week-old male green fluorescent protein (GFP) transgenic C57BL/6 mice were obtained from Beijing Animal Center, China (originally from Jackson Laboratory) and maintained in a pathogen-free animal facility. Experiments were approved by Nankai Animal Care and Use Committee. Chimeric mice of Lrrc19 −/− and WT GFP transgenic C57BL/6 mice were generated basically according to a previously reported method [42] . Briefly, 6-week-old Lrrc19 KO and WT GFP transgenic C57BL/6 mice were lethally irradiated with 9 Gy of total-body irradiation. BM cells were obtained from the femurs of donor mice and collected in RPMI 1640 containing 100 U ml −1 penicillin/streptomycin. Irradiated recipient mice were injected with 200 μl of the appropriated cell suspension via the tail vein. The recipient mice were maintained in a sterile facility for 8 weeks to allow for complete engraftment with donor bone marrow. To assay bone marrow reconstitution, spleens were harvested from chimeric mice, and single-cell suspension of splenocytes were prepared in phosphate-buffered saline (PBS) and then analysed by flow cytometry to detect GFP+ spleen cells and determine donor/recipient chimerism of the hematopoietic compartment. Reagents N-palmitoyl-S-[2,3-bis(palmitoyloxy)-propyl]-(R)-cysteinyl-seryl-(lysyl)3-lysine (Pam3CSK4) and lipopolysaccharide (LPS, 0111B4) were purchased from InvivoGen, San Diego, USA. FITC-labelled LPS and Rhodamine-labelled Pam3CSK4 were from InvivoGen. LRRC19, MyD88, TRIF, IRAK1, IRAK4, TRAF2, TRAF6, TAB2 and TAB3 siRNA and control mocksiRNA were purchased from Ribo, Shenzheng, China. Following antibodies were purchased also, including anti-mouse p38 (Cell Signalling), JNK (Cell Signalling), ERK (Cell Signalling), phosphorylated-p38 (pp38) (Cell Signalling), phosphorylated JNK (pJNK) (Cell Signalling), phosphorylated ERK (pERK) (Cell Signalling), phosphorylated -IκBα (pIkBα) (Cell Signalling), IκBα (ZSGB-Bio), p65 (Santa), LRRC19 (Abcam), V5 (Invitrogen), Myc (Abmart), flag (Abmart), HA (Cell Signalling Technology), ubiquitin (Immunoway), K63-Ub (Enzo), K48-Ub (Cell signalling), TRAF2 (Epitomics), TRAF6 (Santa), MCP-1 (Bioss), MIP-2 (Bioss), Reg3γ (Thermo Scientific), cathelicidin (Abcam), cytokeratin 18 (Invitrogen) and β-actin (Santa); FITC-and PE-conjugated anti-mouse CD11b (ICRF44), anti-Ly6C (ER-MP20) and anti-Ly6G (RB6-8C5) antibodies were purchased from BD Biosciences. Plasmid constructs Plasmids encoding Flag-tagged TLR2, Flag-tagged TLR4, Myc-tagged TRAF2, Myc-tagged TRAF6 and Myc-tagged MyD88 were provided by Dr Chuang (University of California, Berkeley). Plasmids encoding hemagglutinin (HA)-tagged ubiquitin (HA-Ub), hemagglutinin-tagged K48-linked ubiquitin (HA-K48-Ub) and K63-linked ubiquitin (HA-K63-Ub) were obtained from Y. Xiong (University of North Carolina, Chapel Hill). The SEAP (secreted embryonic alkaline phosphatase) reporter plasmids for NF-κB were obtained from Clonetech Laboratories Inc. The murine and human full-length LRRC19, TRAF2 and TRAF6 cDNA clones were obtained from the ATCC. LRRC19 mutants lacking the extracellular domain were constructed by performing PCR with four primers according to a previous method [43] . The PCR products were then ligated into a pcDNA3.1V5/His 6 mammalian expression vector (Invitrogen). All the constructs were confirmed by DNA sequencing (Huada Bio., China). All primers used in this study are listed in Supplementary Table 1(c) . RT–PCR and qRT–PCR Semi-quantitative RT–PCR and quantitative real-time PCR (qRT–PCR) were performed. Briefly, total RNA was extracted from the cells, tissues and organs using TRIzol reagent (Invitrogen Corp). First-strand cDNA was generated from the total RNA using oligo-dT primers and reverse transcriptase (Invitrogen Corp). The PCR products were visualized on 1.0% (wt/vol) agarose gel. Real-time PCR was conducted using QuantiTect SYBR Green PCR Master Mix (Qiagen) and specific primers in an ABI Prism 7000 analyser (Applied Biosystems). GAPDH mRNA expression was detected using each experimental sample as an endogenous control. The fold changes were calculated using the ΔΔC t method according to the manufacturer’s instructions (Applied Biosystems). All the reactions were run in triplicate. Primer sequences are listed in Supplementary Table 1(d) and (e) . In situ hybridization Tissues of mice were fixed in 4% (w/v) paraformaldehyde-fixed and embedded in paraffin according to standard procedures. Briefly, 5 μm sections were deparaffinized, rehydrated through a graded series of ethanol baths, and washed with water treated with 0.1% DEPC three times for 5 min. In situ hybridization of LRRC19 was performed according to the manufacturer’s protocol (TBD sci). Staining was conducted using a diaminobenzidine staining kit. Probes are listed in Supplementary Table 1(f) , were designed based on the published genomic sequences of mouse LRRC19 mRNA (GenBank ID: 224109). Probes were labelled with digoxin (DIG). The sense probes were used as negative controls. Histology and immunostaining For hematoxylin/eosin (H&E) staining, kidneys and bladders were fixed in 10% formalin-buffered saline and embedded in paraffin, 5-μm sections of kidney were cut and stained with H&E. For immunostaining analysis of kidney and bladder tissue, 5-μm-thick sections were prepared from frozen tissue and fixed in acetone (−20 °C) for 10 min. After rehydration in PBS for 5 min and further washing in PBS, tissue sections were blocked with 1% (w/v) BSA and 0.2% (w/v) milk powder in PBS (PBS-BB). The primary antibody was added in PBS-BB and incubated overnight at 4 °C. After PBS washing (three times, 5 min each), tissue was detected with DAB kit or fluorescence labelled second antibody. Nuclei were stained by 4',6-diamidino-2-phenylindole (DAPI). Immunoprecipitation and immunoblotting The cells were lysed with cell-lysis buffer (Cell Signalling Technology), which was supplemented with a protease inhibitor ‘cocktail’ (Calbiochem). The protein concentrations of the extracts were measured using a bicinchoninic acid assay (Pierce). Immunoprecipitation (IP) was performed essentially the same as described by the manufacturer (Thermo Scientific, USA). Cell lysates were preabsorbed with protein A/G agarose beads at 4 °C for 1 h. After centrifuging, the supernatants were incubated with anti-V5 (1: 1,000 dilutions), anti-Myc (1: 1,000 dilutions), anti-TRAF2 (1: 500 dilutions) or anti-TRAF6 (1: 500 dilutions) overnight at 4 °C followed by incubation with protein A/G agarose beads (Santa Cruz Biotechnology) for 2 h at 4 °C. For the immunoblot, hybridizations with primary antibodies were conducted for 1 h at room temperature in blocking buffer. The protein–antibody complexes were detected using peroxidase-conjugated secondary antibodies (Boehringer Mannheim) and enhanced chemiluminescence (Amersham). NF-κB translocation The renal tubular epithelial cells (4 × 10 5 ) were seeded onto coverslips in 24-well dishes and were grown for 24 h before stimulation with E. coli CFT073 (infected) or unstimulated (uninfected) for 3 h, then cells were stained with anti-p65 (D14E12; Cell Signalling) and Alexa Fluor 546–conjugated antibody to rabbit (A-11035; Invitrogen) and then were counterstained for nucleic acids with DAPI. Nuclei were stained with DAPI (blue) (scale bar, 20 μm). NT, nuclear translocation. P65 NT(%)=cellular number with NT/total cellular number. A total of 1 × 10 3 cells per sample were counted. Cells were analysed with a Zeiss LSM 710 laser-scanning confocal microscope. In vitro experiments The human embryo kidney cell line HEK293T cells and HK2 (human renal proximal tubular epithelial cells) were purchased from the American Type Culture Collection (ATCC, USA). HEK293T cells expressing TLR4 (TLR4/CD14/MD2 complexes) and TLR1/2 (TLR1+TLR2) were from IMGENEX, USA. LRRC19 expressing HEK293T cells were prepared by G418 selection after transfecting LRRC19. Primary kidney tubular cells were prepared from kidneys of 2–3-week-old WT and Lrrc19 KO mice and grown in culture according to a standard protocol [44] . Briefly, kidneys from 2–3-week-old mice were rapidly removed under sterile conditions, and minced and digested with a collagenase IV (100 U ml −1 ) in tissue culture medium at 37 °C. Tissue fragments were gently pelleted, washed three times in PBS and then suspended in tissue medium. Cells were plated at a density of 10 6 live cells per ml of cell culture medium and maintained at 37 °C. Cells were confirmed as kidney tubular epithelial cells by staining with anti-cytokeratin antibody. For in vitro stimulation, primary renal tubular epithelial cells or transfected HEK293T cells were washed and stimulated using 5 μg ml −1 Pam3CSK4, 100 ng ml −1 LPS and heat-killed E. coli CFT073 (7.5 × 10 6 CFU) or nonpathogenic DH5α (7.5 × 10 6 CFU, cell: bacteria ratio of 1:25). At the indicated time, culture supernatants were collected and cytokine and bactericidal peptide levels were determined using a commercial ELISA kit (R&D Systems Inc., Wiesbaden- Nordenstadt, Germany). Total RNAs were prepared for transcriptional levels of cytokines and bactericidal peptides. Proteins and the cell lysates were prepared with lysis buffer for immunoblot analyses. For bactericidal analyses by renal tubule epithelial cells, 3 × 10 5 renal tubular epithelial cells from WT and Lrrc19 KO mice in 50 μl of iPIPES (10 mM Pipes, 150 mM NaCl) were stimulated by heat-killed UPEC CFT037 (CFT073, 3 × 10 6 CFU) or DH5α (DH5 α, 3 × 10 6 CFU) for 18 h and then supernatants were collected for bactericidal analyses. The equal number of UPEC CFT037 (1 × 10 3 CFU) were added into WT and Lrrc19 KO supernatants for 3 h. Then supernatants were plated on LB plates for bacteria growth. Killing %=CFU before incubating with supernatants−CFU after incubating with supernatants/CFU before incubating with supernatants In vivo experiments C57BL/6, Tlr4 KO (Nanjing Animal Center, Nanjing, China), Lrrc19 KO and chimeric mice were housed under specific pathogen-free conditions. Tlr4 KO mice were originally obtained from Osaka University, Osaka, Japan. Animal experiments were approved by the Institute’s Animal Ethics Committee of Nankai University. To establish a kidney infection model, anesthetized age-matched (7–8-week-old) female mice were inoculated transurethrally with 5.0 × 10 7 CFU of E. coli CFT073, which are often used in mouse model of renal infection [45] in a volume of 50 μl, and urethras were coated with collodion (Sigma-Aldrich). Six hours post infection, collodion was removed by blotting with acetone. At each time point, organs were homogenized in 1 ml of 0.025% (v/v) Triton X-100/PBS and plated on Lurin-Bertani (LB) agar plates to enumerate CFU. To assess the degree of inflammation, bladders and kidneys were bisected, and one half was either fixed in neutral buffered formalin for histological analysis or quick-frozen in liquid nitrogen for immunostaining analysis. E. coli CFT073 was obtained from the Center of Disease Control in China. For tissue homogenates, tissues were rinsed in ice-cold PBS (0.02 mol l −1 , PH 7.2–7.4). Excess blood was thoroughly removed. Tissues were weighted before homogenization and minced to small pieces and homogenized them in a certain amount of PBS (usually 10 mg tissue to 100 μl PBS.) with a glass homogenizer on ice. The resulting suspension was subjected to ultrasonication or to two freeze–thaw cycles to further break the cell membranes, and after that, centrifugate homogenates for 15 min at 1,500 × g . The specimens were immediately assayed or stored at −20 °C or −80 °C. Enzyme-linked immunosorbent assay Commercial ELISA kits were used to quantitate human IL-8 (Interleukin-8), murine TNFα, IL-6, MCP-1, MIP-2 (R&D Systems) and α-defensin-5 (GENTAUR, CA, USA). The optical density at 450 nm in each sample was measured using a 90 ELISA plate reader. The cytokine levels were quantified from two to three titrations using standard curves. Data analyses Statistical significance of the comparisons between the two groups was determined using a Student’s t -test; whereas the comparisons among the multiple groups were determined using an analysis of variance test. Bacterial counts of kidney tissues between WT and Lrrc19 KO or other mice were analysed by a Mann–Whitney U test. A 95% confidence interval was considered significant and was defined as P <0.05. How to cite this article: Su, X. et al . LRRC19 expressed in the kidney induces TRAF2/6-mediated signals to prevent infection by uropathogenic bacteria. Nat. Commun. 5:4434 doi: 10.1038/ncomms5434 (2014).